Ultra-low-frequency wave-driven diffusion of radiation belt relativistic electrons Van Allen radiation belts are typically two zones of energetic particles encircling the Earth separated by the slot region. How the outer radiation belt electrons are accelerated to relativistic energies remains an unanswered question. Recent studies have presented compelling evidence for the local acceleration by very-low-frequency (VLF) chorus waves. However, there has been a competing theory to the local acceleration, radial diffusion by ultra-low-frequency (ULF) waves, whose importance has not yet been determined definitively. Here we report a unique radiation belt event with intense ULF waves but no detectable VLF chorus waves. Our results demonstrate that the ULF waves moved the inner edge of the outer radiation belt earthward 0.3 Earth radii and enhanced the relativistic electron fluxes by up to one order of magnitude near the slot region within about 10 h, providing strong evidence for the radial diffusion of radiation belt relativistic electrons. The geomagnetic field geometry allows three quasi-periodic motions of outer Van Allen radiation belt [1] relativistic electrons over distinct timescales: gyration about the magnetic field line on a timescale of milliseconds; bounce along the magnetic field line between two magnetic mirror points on a timescale of seconds; drift circling the Earth on a timescale of kiloseconds. Each periodicity gives rise to an approximate constant of motion defined as the adiabatic invariant. Surrounding the highly dynamic outer radiation belt [2] , one outstanding question has been how electrons are accelerated to relativistic energies of several million electron volts. Two invariant-violating processes have been proposed: local acceleration by VLF ( ∼ kHz) chorus waves [3] , [4] and radial diffusion by ULF ( ∼ mHz) waves [5] , [6] , [7] , [8] , [9] . On 30 August 2012, National Aeronautics and Space Administration launched a twin-spacecraft mission, Van Allen Probes (formerly known as the Radiation Belt Storm Probes (RBSP)) [10] , to make the measurements for the identification of acceleration mechanisms. Recent analyses [11] , [12] of the Van Allen Probes data have presented compelling evidence for the local acceleration in the heart of the outer radiation belt. However, the importance of radial diffusion for the radiation belt evolution has not yet been determined definitively. ULF waves have been thought to effectively violate the third adiabatic invariant L * under the drift-resonance condition [5] ω = mω d (with the wave frequency ω , the azimuthal wave mode number m and the electron drift frequency ω d ). The quantity L * is the Roederer’s drift-shell parameter [13] , equal to the equatorial radial distance (made dimensionless by Earth radii R E ) of the adiabatically equivalent electron drift orbit in the dipole field. Violation of the third invariant (but conservation of the first two invariants) causes the radial migration of resonant electrons and consequently the variation of their energies and pitch angles. The electrons in drift resonance with broadband ULF waves move stochastically along the radial direction, which is described by the radial diffusion theory [5] , [7] , [8] . This theory was indirectly supported by the strong correlation between ULF wave power and radiation belt electron flux enhancement [14] , [15] , [16] , [17] , [18] , but due to the limitations in previous particle/field observations, the in situ wave–particle interaction characteristics were lacking to clarify the associated physical process. Particularly, previous works [7] , [14] , [15] , [16] , [19] , [20] often concentrated on the radiation belt reformation events during the geomagnetic storms. These geomagnetic storms did cause marked dynamics of energetic electrons, but the strongly disturbed magnetosphere very likely allowed the concurrence [20] , [21] , [22] of ULF wave-driven radial diffusion and VLF chorus wave-driven local acceleration. The superposition of two processes is not conducive to isolating the contribution of radial diffusion. Here we report a unique radiation belt event serendipitously observed by the Van Allen Probes in the plasmasphere during non-storm times. The plasmasphere is a torus-shaped region of cold and dense plasma surrounding the Earth, where the VLF chorus wave-driven local acceleration seldom occurs. By analysing the high-resolution data and performing the detailed simulation, we demonstrate that the radial diffusion by intense ULF waves was responsible for the radiation belt relativistic electron evolution in this event. Wave modulation of relativistic electrons The radiation belt event of interest occurred on 15 February 2014, with the required particle/field data collected by the Relativistic Electron–Proton Telescope (REPT) [23] and the Magnetic Electron Ion Spectrometer (MagEIS) [24] of the Energetic particle, Composition and Thermal plasma (ECT) instrument suite [25] , the Electric Fields and Waves (EFW) instruments [26] and the Electric and Magnetic Field Instrument Suite and Integrated Science (EMFISIS) instrument suite [27] on board the Van Allen Probes. During the event, the magnetosphere was free from magnetic storms but experienced some weak and short-duration substorms ( Fig. 1a ). 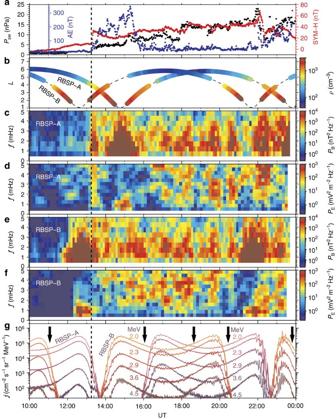Figure 1: An overview of the 15 February 2014 radiation belt event. (a) Solar wind dynamic pressurePsw, geomagnetic activity indices AE (measuring the substorm intensity) and SYM-H (measuring the storm intensity and partially reflecting the variation of solar wind dynamic pressure). (b) Cold electron number densityρfrom the EFW instrument. The density were always beyond 40 cm−3, indicating the locations of Van Allen Probes in the plasmasphere. (c,e) Power spectral densityPBof the compressional ULF wave magnetic field in the MFA coordinate system from the EMFISIS magnetometer. (d,f) Power spectral densityPEof theycomponent ULF wave electric field in the mGSE coordinate system from the EFW instrument. In the outer belt, the ULF wave power were intensified obviously by the solar wind variation after 13:15UT(vertical-dashed line). (g) Spin-averaged differential electron fluxesj(colour-coded according to energy) in the outer radiation belt from the REPT instrument. Black arrows mark the times around which the regular oscillations of fluxes were relatively weak. Such magnetospheric conditions favoured the expansion of plasmasphere to at least L =6.5 ( Figs 1b and 2a,c ; Supplementary Table 1 ). The quantity L is the McIlwain’s drift-shell parameter [28] , equal to the equatorial radial distance (made dimensionless by Earth radii R E ) of the drift orbit of the electron having the same mirror field, second invariant and energy in the dipole field. In the plasmasphere, there were no VLF chorus waves contributing to the local acceleration ( Fig. 2b,d ). In the time range from 13:15 to 24:00 UT , the solar wind dynamic pressure ( Fig. 1a ) exhibited continuous fluctuations especially around 13:15 and 22:00 UT . The solar wind variation drove the generation of ULF waves over a wide frequency range in the outer radiation belt ( Fig. 1c–f ). Correspondingly, the relativistic (2.0–4.5 MeV) electron fluxes oscillated periodically ( Fig. 1g ), which is one of the expected drift-resonance characteristics [29] . In contrast to the previously reported ULF modulation [30] , [31] of electron fluxes at the relatively low energies and/or in a localized spatiotemporal region, this event presented the ULF modulation of highly relativistic electron fluxes for about 10 h throughout the outer radiation belt, serving as an observational evidence for the global and long-lasting drift resonance between ULF waves and relativistic electrons. Figure 1: An overview of the 15 February 2014 radiation belt event. ( a ) Solar wind dynamic pressure P sw , geomagnetic activity indices AE (measuring the substorm intensity) and SYM-H (measuring the storm intensity and partially reflecting the variation of solar wind dynamic pressure). ( b ) Cold electron number density ρ from the EFW instrument. The density were always beyond 40 cm −3 , indicating the locations of Van Allen Probes in the plasmasphere. ( c , e ) Power spectral density P B of the compressional ULF wave magnetic field in the MFA coordinate system from the EMFISIS magnetometer. ( d , f ) Power spectral density P E of the y component ULF wave electric field in the mGSE coordinate system from the EFW instrument. In the outer belt, the ULF wave power were intensified obviously by the solar wind variation after 13:15 UT (vertical-dashed line). ( g ) Spin-averaged differential electron fluxes j (colour-coded according to energy) in the outer radiation belt from the REPT instrument. Black arrows mark the times around which the regular oscillations of fluxes were relatively weak. 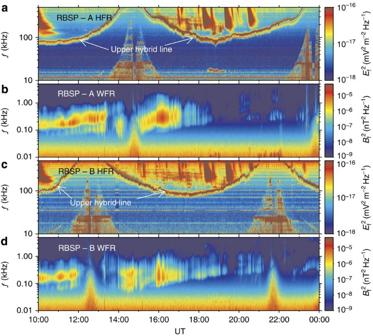Figure 2: Electromagnetic power spectral densities of high-frequency and very-low-frequency waves. (a,c) Wave electric power spectral density from the high-frequency receiver (HFR) of the EMFISIS Suite and Integrated Science suite. The upper hybrid resonance bands (bright lines) had frequencies (positively correlated with the background electron density59) beyond 70 kHz, indicating that the twin spacecrafts stayed in the high-density plasmasphere for the entire orbits. (b,d) Wave magnetic power spectral density from the Waveform Receiver (WFR) of the EMFISIS suite. There were VLF hiss waves in the frequency range 0.1–1.0 kHz contributing to the slow loss of relativistic electrons, but no VLF chorus waves responsible for the local acceleration of relativistic electrons. Full size image Figure 2: Electromagnetic power spectral densities of high-frequency and very-low-frequency waves. ( a , c ) Wave electric power spectral density from the high-frequency receiver (HFR) of the EMFISIS Suite and Integrated Science suite. The upper hybrid resonance bands (bright lines) had frequencies (positively correlated with the background electron density [59] ) beyond 70 kHz, indicating that the twin spacecrafts stayed in the high-density plasmasphere for the entire orbits. ( b , d ) Wave magnetic power spectral density from the Waveform Receiver (WFR) of the EMFISIS suite. There were VLF hiss waves in the frequency range 0.1–1.0 kHz contributing to the slow loss of relativistic electrons, but no VLF chorus waves responsible for the local acceleration of relativistic electrons. Full size image The azimuthal mode number m of ULF waves is required to quantify the drift-resonance process. Wavelet transforms [32] have been performed on the electron fluxes at different energy channels to identify their dominant oscillation periods ( Fig. 3 ). During some time intervals (10:00–13:15, 15:30–16:00, 17:30–19:30, 20:20–21:00 and 23:30–24:00 UT ), the regular oscillations of fluxes were so weak (as marked by the black arrows in Fig. 1g ) that the wavelet transforms mainly captured the power associated with the irregular noise and/or the radial variation of fluxes. Most of the time the dominant oscillation periods of electron fluxes are found to change with energy and location but remain close to the corresponding electron drift periods, which can be considered as the result of the m =1 mode drift-resonance between relativistic electrons and broadband ULF waves [29] , [33] . It should be mentioned that recent magnetohydrodynamic simulation [34] for a magnetic storm had suggested the dominance of m =1 mode ULF waves in the radiation belt region. 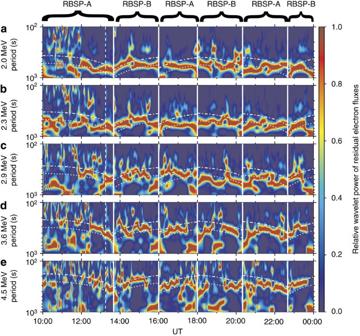Figure 3: Relative wavelet power of residual electron fluxes. (a-e) Relative wavelet power at the energy channels 2.0, 2.3, 2.9, 3.6 and 4.5 MeV, respectively. Residual flux is defined as (j−j0)/j0withjthe spin-averaged differential flux from the REPT instrument andj0the 1,000 s running averagedj, which reflects the oscillation of electron flux at each energy channel. Relative wavelet power is defined as the wavelet power of residual flux normalized by the maximum power with oscillation period <1,000 s. The obtained relative wavelet power (colour-coded scale) of the twin spacecrafts is plotted alternatively to characterize the oscillation of the outer radiation belt electron fluxes. The superposed dotted and dot-dashed lines represent the drift periods of electrons with the equatorial pitch angles 0° and 90° at the corresponding energy channels in the dipole field. The vertical-dashed line denotes the beginning of ULF wave enhancement induced by the solar wind dynamic pressure variation. Figure 3: Relative wavelet power of residual electron fluxes. ( a - e ) Relative wavelet power at the energy channels 2.0, 2.3, 2.9, 3.6 and 4.5 MeV, respectively. Residual flux is defined as ( j − j 0 )/ j 0 with j the spin-averaged differential flux from the REPT instrument and j 0 the 1,000 s running averaged j , which reflects the oscillation of electron flux at each energy channel. Relative wavelet power is defined as the wavelet power of residual flux normalized by the maximum power with oscillation period <1,000 s. The obtained relative wavelet power (colour-coded scale) of the twin spacecrafts is plotted alternatively to characterize the oscillation of the outer radiation belt electron fluxes. The superposed dotted and dot-dashed lines represent the drift periods of electrons with the equatorial pitch angles 0° and 90° at the corresponding energy channels in the dipole field. The vertical-dashed line denotes the beginning of ULF wave enhancement induced by the solar wind dynamic pressure variation. Full size image Global evolution of relativistic electrons The Van Allen Probes passed through the radiation belt six times in the time range of interest. The comparison of the L -dependent electron fluxes observed during each passage is made to identify the global evolution of radiation belt electrons ( Fig. 4 ). Within about 10 h, the inner edge of the outer belt moved inward about 0.3 R E at 2.0 MeV and 0.8 R E at 4.5 MeV. Around the inner edge, the electron fluxes increased by an average factor of up to 10. To exclude the possible adiabatic effect associated with the compression of magnetosphere, these electron fluxes are transformed into phase space density (PSD) in the adiabatic invariant coordinate system ( Fig. 5a ; Supplementary Figs 1–3 ; Supplementary Note 1 ). For the fixed L * near the slot region, the variation of mapped L with time was below 0.05 throughout the event ( Fig. 6 ). The initial PSD peaked at the large L * (that is, the external source region) and monotonically decreased with the decreasing L *. As time went on, the external source showed some fluctuations. At the centre of the outer belt ( L *≈4.3), the PSD remained unchanged, once again demonstrating the absence of local acceleration. In the slot region, the inner edge of the outer belt was transported inward about 0.3 R E . Specifically, at L *≈3.6, the PSD gradually increased by one order of magnitude within 10 h. These global evolution characteristics were qualitatively consistent with the prediction of radial diffusion theory [35] , [36] . It should be mentioned that the very strong fluctuations of electron PSDs after 22:00 UT were perhaps associated with the coherent transport process [33] . 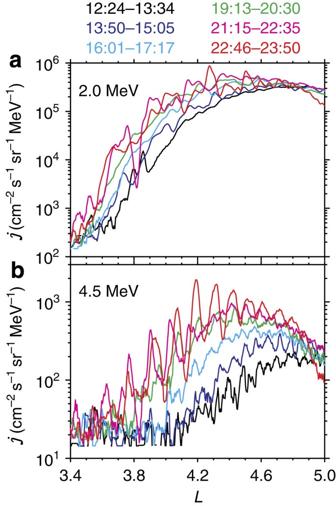Figure 4: Radial profiles of relativistic electron fluxes for six outer radiation belt passages. Each colour-coded profile shows theL-dependent differential fluxjfrom REPT instrument during a passage. (a,b) Differential fluxes of electrons with the equatorial pitch angles 55° at the energy channels 2.0 and 4.5 MeV, respectively. Because of the latitudinal variation of twin spacecrafts, the corresponding local pitch angles varied between 55° and 90° in the TS04D geomagnetic field model60. Electron fluxes at the other energy channels 2.3, 2.9 and 3.6 MeV exhibited the similar characteristics. Figure 4: Radial profiles of relativistic electron fluxes for six outer radiation belt passages. Each colour-coded profile shows the L -dependent differential flux j from REPT instrument during a passage. ( a , b ) Differential fluxes of electrons with the equatorial pitch angles 55° at the energy channels 2.0 and 4.5 MeV, respectively. Because of the latitudinal variation of twin spacecrafts, the corresponding local pitch angles varied between 55° and 90° in the TS04D geomagnetic field model [60] . Electron fluxes at the other energy channels 2.3, 2.9 and 3.6 MeV exhibited the similar characteristics. 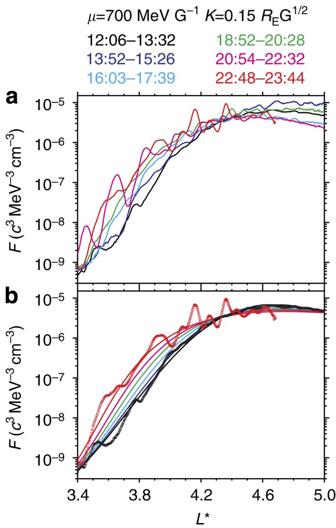Figure 5: Radial profiles of relativistic electron phase space densities for six outer radiation belt passages. Each colour-coded profile shows theL*-dependent phase space densityFat the fixed first adiabatic invariantμ=700 MeV G−1and second adiabatic invariantK=0.15REG1/2during a passage. The corresponding energies were about 1.0 MeV atL*=5.5 and 2.5 MeV atL*=3.4, and the corresponding local pitch angles were 40°–70°. (a) Observations (lines) from MagEIS and REPT instruments in the TS04D geomagnetic field model. (b) Simulations (lines) from the radial diffusion equation, overplotted with the observations (circles) for ease of comparison. Full size image Figure 5: Radial profiles of relativistic electron phase space densities for six outer radiation belt passages. Each colour-coded profile shows the L *-dependent phase space density F at the fixed first adiabatic invariant μ =700 MeV G −1 and second adiabatic invariant K =0.15 R E G 1/2 during a passage. The corresponding energies were about 1.0 MeV at L *=5.5 and 2.5 MeV at L *=3.4, and the corresponding local pitch angles were 40°–70°. ( a ) Observations (lines) from MagEIS and REPT instruments in the TS04D geomagnetic field model. ( b ) Simulations (lines) from the radial diffusion equation, overplotted with the observations (circles) for ease of comparison. 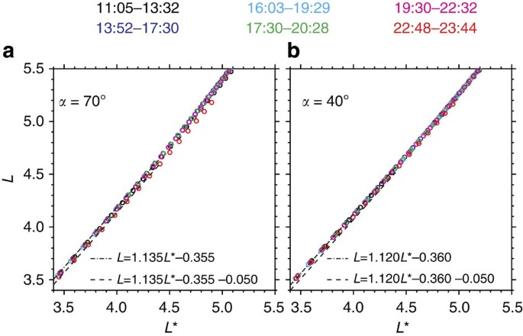Figure 6: Mapping relations betweenLandL* for six outer radiation belt passages. Mapping relations (circles colour-coded according to the time) are calculated every 300 s in the TS04D geomagnetic field model. (a,b) Mapping relations at two different local pitch angles 70° and 40°, respectively. The dot-dashed and dashed lines are overplotted to identify the variation of the mappedLwith time for the fixedL* near the slot region. Similar characteristics can be found in the mapping relations at the other local pitch angles. Full size image Figure 6: Mapping relations between L and L * for six outer radiation belt passages. Mapping relations (circles colour-coded according to the time) are calculated every 300 s in the TS04D geomagnetic field model. ( a , b ) Mapping relations at two different local pitch angles 70° and 40°, respectively. The dot-dashed and dashed lines are overplotted to identify the variation of the mapped L with time for the fixed L * near the slot region. Similar characteristics can be found in the mapping relations at the other local pitch angles. Full size image The radial diffusion of radiation belt electrons is simulated by solving the equation [37] with the electron PSD F and the radial diffusion rate D L*L* calculated from the observed ULF waves [9] ( Fig. 7 ). The simulations ( Fig. 5b ; Supplementary Fig. 4 ; Supplementary Note 2 ) well reproduce the average rate and extent of the observed PSD variations. The radial diffusion process can effectively reduce the electron PSD gradients [35] . In the region L *>4.3, the electron PSD behaved smoothly and consequently presented minor changes. In contrast, the electron PSD possessed a very steep gradient in the region L *<4.3 and then allowed the significant enhancement. 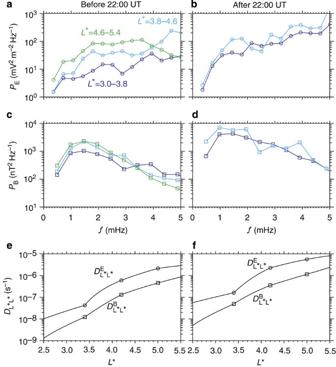Figure 7: Electromagnetic power spectral densities of ultra-low-frequency waves and radial diffusion rates. (a–d) Averaged electricPE(circles) and magneticPB(squares) power spectral densities in three different regions before and after 22:00UT. Solid lines are introduced to guide the eye. (e,f) Radial diffusion rates (lines) from the electricand magneticperturbations. Symbols are drawn to mark the diffusion rates at the centres of the three spatial regions. The total radial diffusion rateswere the sum of the electric and magnetic radial diffusion rates. Figure 7: Electromagnetic power spectral densities of ultra-low-frequency waves and radial diffusion rates. ( a – d ) Averaged electric P E (circles) and magnetic P B (squares) power spectral densities in three different regions before and after 22:00 UT . Solid lines are introduced to guide the eye. ( e , f ) Radial diffusion rates (lines) from the electric and magnetic perturbations. Symbols are drawn to mark the diffusion rates at the centres of the three spatial regions. The total radial diffusion rates were the sum of the electric and magnetic radial diffusion rates. Full size image There was an average enhancement of relativistic electron fluxes by up to one order of magnitude within about 10 h on 15 February 2014, which could be easily misinterpreted in the framework of the VLF chorus wave-driven local acceleration. The high-resolution data and the detailed simulation clearly show that, in the absence of VLF chorus waves, the ULF waves could radially diffuse and effectively accelerate the radiation belt electrons in this event. The ULF waves [38] , [39] , [40] , [41] , [42] , [43] , [44] , as well as the VLF chorus waves [45] , [46] , [47] , [48] , [49] , [50] , [51] , [52] , [53] , [54] , are commonly observed in the magnetosphere. To provide a more comprehensive picture, we additionally analyse two more radiation belt events with the concurrence of ULF and VLF chorus waves ( Supplementary Figs 5–14 ; Supplementary Tables 2 and 3 ; Supplementary Note 3 ). During the 18 January 2013 event, there were moderate ULF waves but quite weak VLF chorus waves. The radial diffusion, dominating over the local acceleration, caused the earthward movement of the inner edge of the outer radiation belt. In contrast, both moderate ULF waves and strong VLF chorus waves occurred during the 22 September 2014 event. The local acceleration produced the relativistic electron PSD peaks, and the radial diffusion redistributed the electrons along the radial direction to reduce the PSD gradients. Our results present evidence for the importance of ULF wave-driven radial diffusion in the outer radiation belt dynamics. Under differing magnetospheric conditions, the accurate contributions of local acceleration and radial diffusion to the radiation belt evolution should be carefully examined. The radial diffusion can play a dominant role in some radiation belt electron acceleration events (such as the one discussed here). Compared with the local acceleration in the previously reported marked events [11] , [12] , [21] , the radial diffusion in the present event yielded a smaller acceleration rate and a smaller relativistic electron flux enhancement. However, no matter how strong the action of local acceleration is, the additional redistribution of relativistic electrons by the radial diffusion would constitute an important part of the outer radiation belt dynamics [11] , [33] , [35] , [55] , [56] , [57] . Calculation of wave power spectral density We use the level-3 magnetic field data with the time resolution of 1 s in the Geocentric Solar Magnetospheric coordinate system to obtain the magnetic power spectral density of ULF waves. A three-step procedure is performed as follows. First, the magnetic field data are running averaged over 11 s to reduce the spin modulation of Van Allen Probes [44] . Then, these magnetic field data are projected on the so-called mean field aligned (MFA) coordinates [58] . In the MFA coordinate system, the parallel direction is determined by the 2,048-s running average of the instantaneous magnetic field, the azimuthal direction is obtained by the cross product of the parallel vector and the satellite position vector, and the radial direction completes the triad. This system is used to separate magnetic field perturbations into the toroidal (azimuthal), poloidal (radial) and compressional (parallel) components [26] . Finally, an overlapped (80%) 2,048-point fast Fourier transform is adopted to calculate the power spectral densities of each magnetic field components. The obtained power spectra densities have the time resolution of 6.83 min and the frequency resolution of 0.49 mHz. We use the level-3 electric field data with the time resolution of 10.9 s in the modified geocentric solar ecliptic (mGSE) coordinate system to obtain the electric power spectral density of ULF waves. The mGSE unit vectors ( X mGSE , Y mGSE and Z mGSE ) can be generally expressed in terms of the GSE unit vectors ( X GSE , Y GSE and Z GSE ) and the spin axis unit vector S GSE : X mGSE = S GSE , , and Z mGSE = X mGSE × Y mGSE . When the spin axis points towards the sun ( S GSE = X GSE ), the mGSE system is exactly the same as the GSE system. The EFW instrument only measured the two electric field components in the spin plane, and the third component has to be derived from the assumption E · B =0. For this event after 22:00 UT , the magnetic field component B x of RBSP-B in the mGSE system was nearly zero and the electric field component E x was unconstrained by the E · B =0 condition, not allowing the calculation of electric field vectors in the MFA system. Note that the most significant ULF waves happened to be generated after 22:00 UT . Hence, we calculate the power spectral densities of the electric field components in the mGSE system (rather than in the MFA system) to ensure the continuous monitoring of ULF waves throughout this event. Specifically, an overlapped (80%) 256-point fast Fourier transform is performed on the electric field data (with the preliminary substraction of the co-rotation electric field and the V sc × B electric field induced by the satellite motion through the Earth’s magnetic field), and the obtained the electric field power spectral densities possess the time resolution of 9.3 min and the frequency resolution of 0.36 mHz. It should be mentioned the power spectral densities exhibited unphysical intensification [44] associated with the steep variation of the background magnetic field during the averaging time of 2,048 s in the region L <3 or the contamination by the large V sc × B electric field in the region L <2.5. Calculation of radial diffusion rates The radial diffusion is generally produced by both the ULF electric and magnetic perturbations. In this event, the m =1 mode symmetric drift resonance is suggested to be dominant. The corresponding radial diffusion rates are written as [9] with the equatorial magnetic field magnitude at the Earth’s surface B 0 =0.312 G, the Lorentz factor of electrons γ , the Earth’s radii R E , and the power spectral densities of the azimuthal wave electric field P E and the compressional wave magnetic field P B at the resonant frequency ω = ω d in the MFA system. As discussed in the previous section, the azimuthal wave electric field cannot be obtained continuously. In this study, P E in the MFA system is approximated as the power spectral density of the y component electric field in the mGSE system. We calculate the radial diffusion rates in two time ranges (14:00–22:00 and 22:00–24:00 UT ). In each time range, we average the wave power in three spatial regions ( L *=3.4±0.4, 4.2±0.4 and 5.0±0.4) and then obtain the L *-dependent ULF wave power distribution through the linear interpolation. In the inner region L *<3.4, the wave power is assumed to equal that at L *=3.4; in the outer region L *>5.0 before 22:00 UT or L *>4.2 after 22:00 UT , the wave power is assumed to equal that at L *=5.0 or 4.2. Note that there were no ULF wave data in the region L *=5.0±0.4 after 22:00 UT . These assumptions would not significantly affect our conclusions, since the ULF wave-driven variation in electron PSDs mainly occurred in the region L *=3.4–4.2. In the frequency range 1–5 mHz, the obtained electromagnetic power spectral densities ( Fig. 7a–d ) were comparable to the previous statistical results [38] , [39] , [40] , [41] , [43] . The obtained electric diffusion rates dominated over the magnetic diffusion rates ( Fig. 7e,f ), consistent with the previous calculations [38] , [40] , [43] . Simulation of radiation belt evolution The simulation code is extracted from our previously developed STEERB model [37] . The fully implicit finite difference method is adopted to solve the radial diffusion equation with the computational domain 2.5≤ L *≤5.5. The initial condition is given by the observed electron PSD during the first passage (12:06–13:32 UT ) of the outer radiation belt. The electron PSD is assumed to be fixed at the outer boundary L *=5.5 and to be zero at the inner boundary L *=2.5. Software availability The software for wavelet analysis is available at http://paos.colorado.edu/research/wavelets/ . How to cite this article: Su, Z. et al. Ultra-low-frequency wave-driven diffusion of radiation belt relativistic electrons. Nat. Commun. 6:10096 doi: 10.1038/ncomms10096 (2015).